eIF1A augments Ago2-mediated Dicer-independent miRNA biogenesis and RNA interference MicroRNA (miRNA) biogenesis and miRNA-guided RNA interference (RNAi) are essential for gene expression in eukaryotes. Here we report that translation initiation factor eIF1A directly interacts with Ago2 and promotes Ago2 activities in RNAi and miR-451 biogenesis. Biochemical and NMR analyses demonstrate that eIF1A binds to the MID domain of Ago2 and this interaction does not impair translation initiation. Alanine mutation of the Ago2-facing Lys56 in eIF1A impairs RNAi activities in human cells and zebrafish. The eIF1A–Ago2 assembly facilitates Dicer-independent biogenesis of miR-451, which mediates erythrocyte maturation. Human eIF1A (heIF1A), but not heIF1A(K56A), rescues the erythrocyte maturation delay in eif1axb knockdown zebrafish. Consistently, miR-451 partly compensates erythrocyte maturation defects in zebrafish with eif1axb knockdown and eIF1A(K56A) expression, supporting a role of eIF1A in miRNA-451 biogenesis in this model. Our results suggest that eIF1A is a novel component of the Ago2-centred RNA-induced silencing complexes (RISCs) and augments Ago2-dependent RNAi and miRNA biogenesis. MicroRNAs (miRNAs) are ∼ 22-nucleotide (nt) endogenous noncoding RNAs involved in gene expression regulation. Their genes are usually transcribed by RNA polymerase II or III [1] , [2] . The resulting primary miRNAs contain characteristic hairpins, which are excised in the nucleus by Drosha/DGCR8 to yield the pre-miRNAs [3] , [4] . Subsequently, the Exportin-5/Ran-GTP complex translocates the pre-miRNAs to the cytoplasm [5] , [6] , where they are engaged by DICER to form a RISC loading complex. The RISC loading complex includes TRBP and Ago2 (refs 7 , 8 , 9 ), while ADAR1 facilitates pre-miRNA loading [10] . In the canonical miRNA biogenesis pathway, DICER removes the terminal loop region to yield mature miRNA [11] , [12] , [13] . Recent studies revealed that miR-451 is produced by an alternative DICER-independent pathway, where pre-miR-451 is loaded directly onto Ago2 and sliced on the 3′-hairpin arm, as guided by the 5′-end of the hairpin, yielding a 30-nt cleaved species [14] , [15] , [16] . A 3′-resection activity by PARN trims ∼ 7 nt to produce the 23-nt miR-451 (ref. 17 ). However, the mechanisms of DICER-independent miRNA biogenesis have remained elusive. miRNAs are incorporated into effector ribonucleoprotein complexes called RNA-induced silencing complexes (RISCs) to exert RNA interference (RNAi). RISCs can suppress translation without messenger RNA (mRNA) degradation, destabilize mRNAs by deadenylation or directly degrade mRNAs by Ago2 slicer activity [12] , [18] , [19] , [20] and inhibit translation at the stage of initiation or elongation [21] , [22] . The core of RISCs is a member of the Ago protein family [23] . In mammals, this family consists of four members (Ago1–4). Although these four Ago proteins can suppress translation of their target mRNAs, only Ago2 (also known as eIF2C2) is endonucleolytically active [19] , [20] . Ago2 is composed of four globular domains (GDs) (N, PAZ, MID and PIWI) and two structured linker domains (L1 and L2) [24] . MID and PAZ domains harbour the 5′-phosphate and 3′-hydroxyl termini of miRNA, respectively [25] , [26] , while the PIWI domain is responsible for the cleavage–slicer activity [27] , [28] . Crystal structures of human Ago2 revealed that the 5′-end of miRNA is tethered to Argonaute through interactions with a binding pocket that is mostly formed by the MID domain [29] , [30] . Eukaryotic translation initiation factor eIF1A is composed of a GD and two unstructured tails (N- and C-terminal tails), which are absent in prokaryotic initiation factor-1 (IF1). The eIF1A-GD consists of an IF homologous oligonucleotide/oligosaccharide-binding fold, and an additional subdomain C-terminal to the oligonucleotide/oligosaccharide-binding fold that contains two alpha helices and two extended strands, which pack to the helix on opposite sites. The GD contains a large RNA-binding face [31] , which is directed towards the ribosome [32] , [33] Here we find that the GD of eIF1A, which is conserved from IF1 to eIF1A, directly binds to Ago2, and that the MID domain of Ago2 interacts with eIF1A but does not affect eIF1A’s function in translation initiation. eIF1A forms a complex with Ago2 and promotes Ago2 cleavage activity in RNAi, and enhances Ago2 activity in miR-451 production in human cells and the developing zebrafish. The results support the notion that eIF1A is a component of the Ago2-centred RISCs. eIF1A interacts with Ago2 To identify new components of the protein networks that participate in DICER-independent miRNA biogenesis and Ago2-mediated RNAi, we generated a human embryonic kidney 293 (HEK293) cell line that stably expresses Flag-HA (haemagglutinin)-Ago2 for immunoprecipitation analyses. Eukaryotic translation initiation factor eIF1A is a previously unrecognized Ago2-interaction protein that is immunoprecipitated by Ago2 in cell lysates and colocalizes with Ago2 in mammalian cells ( Fig. 1a,b ). To test the specificity of the eIF1A–Ago interaction, we tested for possible interactions with other members of the Ago family using HEK293 cells stably expressing Ago 1–4 (ref. 34 ). Transiently overexpressed eIF1A showed interaction with Ago2, but not Ago1, Ago3 or Ago4 ( Fig. 1c ). 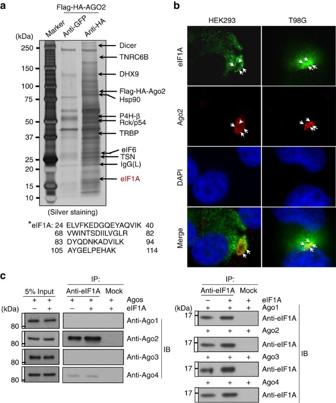Figure 1: eIF1A interacts with Ago2. (a) Proteins co-immunoprecipitated with Flag-HA-Ago2 from HEK293 cells were separated by SDS–polyacrylamide gel electrophoresis (silver staining) and analysed by mass spectrometry. eIF1A is a novel Ago2-interacting protein (* indicates the detected peptides of eIF1A). (b) Fluorescence immunostaining was performed with anti-eIF1A (monoclonal) and anti-Ago2 (monoclonal) antibodies and DAPI (4′,6-diamidino-2-phenylindole) in HEK293 and human glioblastoma multiforme T98G cells. White arrows show the co-localized eIF1A and Ago2. (c) eIF1A interacts with Ago2. HumaneIF1Awas transiently overexpressed in stable HEK293 cells stably expressing Agos (1∼4). Immunoprecipitation assays were performed with anti-eIF1A (monoclonal) antibody and immunoblotting (IB) with anti-Agos antibodies in the upper panel and anti-eIF1A antibodies in the lower panel. Figure 1: eIF1A interacts with Ago2. ( a ) Proteins co-immunoprecipitated with Flag-HA-Ago2 from HEK293 cells were separated by SDS–polyacrylamide gel electrophoresis (silver staining) and analysed by mass spectrometry. eIF1A is a novel Ago2-interacting protein (* indicates the detected peptides of eIF1A). ( b ) Fluorescence immunostaining was performed with anti-eIF1A (monoclonal) and anti-Ago2 (monoclonal) antibodies and DAPI (4′,6-diamidino-2-phenylindole) in HEK293 and human glioblastoma multiforme T98G cells. White arrows show the co-localized eIF1A and Ago2. ( c ) eIF1A interacts with Ago2. Human eIF1A was transiently overexpressed in stable HEK293 cells stably expressing Agos (1 ∼ 4). Immunoprecipitation assays were performed with anti-eIF1A (monoclonal) antibody and immunoblotting (IB) with anti-Agos antibodies in the upper panel and anti-eIF1A antibodies in the lower panel. Full size image eIF1A binds to Ago2 in an RNA-independent manner To identify which of the individual domain(s) of Ago2 interacts with eIF1A, we examined the interaction of recombinant—RNase A and Benzonase-treated—L1,PAZ, MID and PIWI domains of Ago2 with glutathione S -transferase (GST)-tagged eIF1A in pull-down assays. RNA-free eIF1A specifically interacted with the RNA-free MID domain ( Fig. 2a ; Supplementary Fig. 1a ). To further characterize the interaction between human eIF1A fragments and Ago2, we screened recombinant GST-tagged eIF1A and eIF1A mutants (N-tail deletion (ND), C-tail deletion and GD, Supplementary Fig. 1b,c ) for interaction with Ago2. GST-tagged full-length, ND, C-tail deletion (CD) and GD of eIF1A interacted with Ago2 but not the GST-tag alone, indicating that the eIF1A-GD is required and sufficient for the interaction with Ago2 ( Fig. 2b ). We further investigated the interaction between RNase A and Benzonase-treated eIF1A and the MID domain by nuclear magnetic resonance (NMR) spectroscopy. The Unlabelled, Sumo-tagged MID domain titrated into a 15 N-labelled sample of eIF1A at molar ratio of 1:1 (eIF1A:SMT3-MID) ( Fig. 2c ) resulted in broadening of eIF1A resonances characteristic of the complex being in an intermediate exchange regime. The resonances of the eIF1A-GD experience more broadening when compared with the unstructured tails. For instance, resonances of Val55, Lys56 and Lys67 residues of 15 N-eIF1A-GD show broadening upon MID domain titration ( Fig. 2c ). These results suggest that the interaction of eIF1A and Ago2 primarily involves the GD of eIF1A. Furthermore, when unlabelled RNA-free eIF1A was titrated to the RNA-free 15 N-MID domain at molar ratio of 1:1, we observed broadening of the MID resonances indicative of direct binding between the two proteins ( Fig. 2d ). We verified that eIF1A does not bind to the SMT3-tag (strong signals in Fig. 2d ). These NMR data demonstrate that eIF1A directly interacts with Ago2 in an RNA-independent manner. 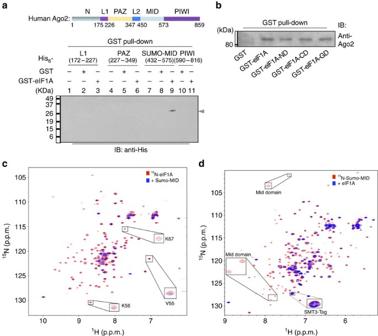Figure 2: eIF1A binds to the MID domain of Ago2 in a RNA-binding-independent manner. (a) Human eIF1A interacts with the MID fragment of human Ago2. Recombinantly expressed and Benzonase-treated Ago2 fragments and recombinantly expressed GST-eIF1A were used for GST pull-down analyses followed by western blotting with anti-His antibodies (IB, immunoblotting). The arrow shows that the MID fragment interacts with eIF1A. (b) The globular domain (GD) of eIF1A interacts with Ago2. Recombinantly expressed and Benzonase-treated GST, GST-eIF1A and mutants (ND, 25∼144 aa; CD, 1∼114 aa; GD, 25∼114 aa) were used for GST pull-down assays with cell lysates of HEK293 stably expressing Ago2. (c)1H–15N transverse relaxation optimized spectroscopy (TROSY)–heteronuclear single-quantum coherence (HSQC) spectrum of15N-eIF1A titrated with the Sumo-MID (432∼575 aa). The titration of RNA-free-Sumo-MID leads to broadening of RNA-free15N-eIF1A resonances (molar ratio of 1:1). Inserted frames show the broadening of resonances of V55, K56 and K67 residues in eIF1A upon MID titration. (d)1H–15N TROSY–HSQC spectrum of15N-Sumo-MID titrated with eIF1A. The titration of eIF1A (molar ratio of 1:1) results in broadening1H–15N TROSY–HSQC crosspeaks coming from the15N-MID domain, but not from15N-Sumo (SMT3) tag. Inserted frames show the broadening of resonances of residues from the MID domain, but not from SMT3-Tag (SUMO-tag), upon eIF1A titration. Figure 2: eIF1A binds to the MID domain of Ago2 in a RNA-binding-independent manner. ( a ) Human eIF1A interacts with the MID fragment of human Ago2. Recombinantly expressed and Benzonase-treated Ago2 fragments and recombinantly expressed GST-eIF1A were used for GST pull-down analyses followed by western blotting with anti-His antibodies (IB, immunoblotting). The arrow shows that the MID fragment interacts with eIF1A. ( b ) The globular domain (GD) of eIF1A interacts with Ago2. Recombinantly expressed and Benzonase-treated GST, GST-eIF1A and mutants (ND, 25 ∼ 144 aa; CD, 1 ∼ 114 aa; GD, 25 ∼ 114 aa) were used for GST pull-down assays with cell lysates of HEK293 stably expressing Ago2. ( c ) 1 H– 15 N transverse relaxation optimized spectroscopy (TROSY)–heteronuclear single-quantum coherence (HSQC) spectrum of 15 N-eIF1A titrated with the Sumo-MID (432 ∼ 575 aa). The titration of RNA-free-Sumo-MID leads to broadening of RNA-free 15 N-eIF1A resonances (molar ratio of 1:1). Inserted frames show the broadening of resonances of V55, K56 and K67 residues in eIF1A upon MID titration. ( d ) 1 H– 15 N TROSY–HSQC spectrum of 15 N-Sumo-MID titrated with eIF1A. The titration of eIF1A (molar ratio of 1:1) results in broadening 1 H– 15 N TROSY–HSQC crosspeaks coming from the 15 N-MID domain, but not from 15 N-Sumo (SMT3) tag. Inserted frames show the broadening of resonances of residues from the MID domain, but not from SMT3-Tag (SUMO-tag), upon eIF1A titration. Full size image Ago2 interaction does not impair eIF1A translation functions On the basis of the observed spectral changes ( Fig. 2c ), we generated three eIF1A mutants: V55A, K56A and K67A. To test whether the mutants are folded, we recorded a transverse relaxation optimized spectroscopy–heteronuclear single-quantum coherence spectrum of eIF1A K56A . The spectrum clearly shows that eIF1A K56A is properly folded ( Supplementary Fig. 2 ). To examine the roles of Val55, Lys56 and Lys67 of eIF1A in full-length eIF1A–Ago2 interaction, we generated HEK293 cell lines stably expressing single eIF1A mutants (V55A, K56A or K67A) involved in Ago2–eIF1A interaction. As determined by immunoprecipitation, all three mutations reduced eIF1A–Ago2 interaction ( Fig. 3a ), suggesting that these amino acids in eIF1A are important for the interaction between Ago2 and full-length eIF1A. In an in vitro dual-luciferase translation assay, elevated eIF1A K56A increases cap-dependent and IRES-dependent translation, to a similar degree as wild-type eIF1A ( Fig. 3b ), suggesting that the K56A mutation does not compromise the activity of eIF1A in translation initiation. In addition, eIF1A K56A does not repress polysome complex formation activities in polysome profiling analyses ( Fig. 3c ), indicating that the K56A mutation does not generally impair translation. Taken together, these data suggest that eIF1A directly interacts with Ago2 in an RNA-binding-independent manner, the MID domain of Ago2 binds to the GD of eIF1A and that the interaction between eIF1A and Ago2 does not impair eIF1A functions in translation initiation. 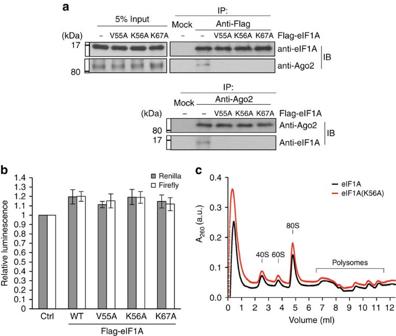Figure 3: Lys56 in eIF1A is important for full-length eIF1A–Ago2 interaction, but K56A mutation in eIF1A does not impair translation initiation. (a) Immunoprecipitation (IP) assays were performed with anti-Flag antibodies in HEK293 cell lines stably expressing Flag-tagged eIF1A and eIF1A mutants. Bottom panel: immunoprecipitation assays were performed with anti-Ago2 antibodies. Immunoblotting (IB) assays were performed with anti-eIF1A and anti-Ago2 antibodies. (b) 0.3 μg added purified Flag-eIF1A (K56A) mutants per reaction display similar promotion effects as 0.3 μg added purified Flag-eIF1A and Flag-eIF1A mutants per reaction in cap-dependent and IRES-dependent translation in dual-luciferase assaysin vitro. Relative luminescence results are shown. Three independent experiments were performed (mean±s.d.,n=3). (c) Polysome profiling analyses with HEK293 cell lines stably expressing eIF1A or eIF1A (K56A). Extracts of the indicated cell lines were subjected to sucrose density gradient centrifugation. The ribosome profiles (recorded at 260 nm) and the positions of the 40S/60S ribosomal subunits, 80S monosome and polyribosomes are shown. WT, wild type. Figure 3: Lys56 in eIF1A is important for full-length eIF1A–Ago2 interaction, but K56A mutation in eIF1A does not impair translation initiation. ( a ) Immunoprecipitation (IP) assays were performed with anti-Flag antibodies in HEK293 cell lines stably expressing Flag-tagged eIF1A and eIF1A mutants. Bottom panel: immunoprecipitation assays were performed with anti-Ago2 antibodies. Immunoblotting (IB) assays were performed with anti-eIF1A and anti-Ago2 antibodies. ( b ) 0.3 μg added purified Flag-eIF1A (K56A) mutants per reaction display similar promotion effects as 0.3 μg added purified Flag-eIF1A and Flag-eIF1A mutants per reaction in cap-dependent and IRES-dependent translation in dual-luciferase assays in vitro . Relative luminescence results are shown. Three independent experiments were performed (mean±s.d., n =3). ( c ) Polysome profiling analyses with HEK293 cell lines stably expressing eIF1A or eIF1A (K56A). Extracts of the indicated cell lines were subjected to sucrose density gradient centrifugation. The ribosome profiles (recorded at 260 nm) and the positions of the 40S/60S ribosomal subunits, 80S monosome and polyribosomes are shown. WT, wild type. Full size image eIF1A promotes Ago2-mediated miRNA-guided RNAi in vitro To examine whether eIF1A plays a role in Ago2-mediated RNAi, we employed a human HMGA2 3′-untranslated region (UTR) mutant that harbours a characterized native let-7 target site [35] ( Fig. 4a ). This assay evaluates the dependence of eIF1A and its mutants on let-7a/Ago2-mediated cleavage of the target mRNA. In the RNAi in vitro assay reactions with added eIF1A or eIF1A mutants without Ago2, no cleavage product was observed, suggesting that the cleavage is Ago2 dependent ( Fig. 4b ). Interestingly, we found that high concentrations of eIF1A increased HMGA2 3′-UTR mutant cleavage, while eIF1A mutants (V55A, K56A and K67A) significantly reduced the level of cleavage products ( Fig. 4b,c ), indicating that eIF1A augments Ago2-mediated RNAi activities in vitro . To investigate the effects of eIF1A in Ago2-mediated miRNA-guided RNAi activities in cells, we used green fluorescent protein (GFP) reporters containing let-7-targeted sequences [36] . Because transient knockdown of eIF1A in HEK293 cells led to significant decrease of cell viability ( Supplementary Fig. 3 ), we employed specific eIF1A–Ago2 interaction interference with eIF1A K56A . Increased eIF1A levels elevated let-7 RISC activity, while eIF1A (K56A) mutant compromised let-7 RISC activity ( Fig. 4d,e ). Elevated eIF1A and Ago2 decrease cellular GFP mRNA levels as determined by quantitative (q)PCR ( Fig. 4f ). In contrast, eIF1A K56A caused increased cellular GFP mRNA levels ( Fig. 4f ). These results suggest that eIF1A forms a complex with Ago2 and promotes Ago2-mediated RNAi in human cells in vitro . 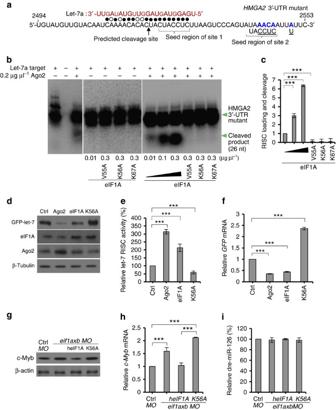Figure 4: eIF1A augments Ago2-mediated RNAi. (a) Sequence of the humanHMGA23′-UTR fragment mutant with two native let-7 target sites. Filled circles: Watson–Crick complementarity; open circles: non-Watson–Crick complementarity. Mutated nucleotides are shown in blue and wild-type nucleotides were underlined (to neutralize site 2 and to reduce self-complementarity). (b)In vitroeffects of eIF1A on Ago2-mediated RNA cleavage. eIF1A or the indicated mutants were incubated with Ago2, synthetic let-7a and 5′-32P end-labelledHMGA23′-UTR mutants. RNAs were analysed by northern blot and autoradiographs analyses. (c) Statistical analyses of three independentin vitroassays inb. (d) Western blot assays of effects of eIF1A and eIF1A (K56A) mutant on GFP-let-7 reporter expression. Ago2, eIF1A or eIF1A (K56A) were transiently overexpressed in HEK293 cells stably expressing reporter GFP-let-7. (e)The expression ratio between tubulin and GFP reporter in the same gel were calculated. Intact (100%) RISC activity was considered in control cells. The relative RISC activities under overexpression conditions of the indicated genes or mutants were obtained by comparison with the control. (f) RelativeGFPreporter mRNAs indby quantitative real-time PCR (qPCR). (g) Western blot assays of zebrafish c-Myb in the indicated zebrafish groups at 28 h.p.f. (control,eif1axbMO (62.5 μM, 1 nl),eif1axbMO (62.5 μM, 1 nl) plus human eIF1A (heIF1A) (mRNA, 1 μg μl−1, 1,000 pl) andeif1axbMO (62.5 μM, 1 nl) plus heIF1A (K56A) mutant (mRNA, 1 μg μl−1, 1,000 pl)). Proteins were extracted from >10 zebrafish per group. (h) Relativec-MybmRNAs in each group ingby qPCR. Total RNAs were extracted from >10 zebrafish per group. (i) Taqman PCR assays of relative zebrafish miR-126 (dre-miR-126) in each group ing. Total RNAs were extracted from >10 zebrafish per group. In all statistical comparisons, three independent experiments were performed (mean±s.d.,n=3 experiments, Student’st-test). ***P<0.01. Figure 4: eIF1A augments Ago2-mediated RNAi. ( a ) Sequence of the human HMGA2 3′-UTR fragment mutant with two native let-7 target sites. Filled circles: Watson–Crick complementarity; open circles: non-Watson–Crick complementarity. Mutated nucleotides are shown in blue and wild-type nucleotides were underlined (to neutralize site 2 and to reduce self-complementarity). ( b ) In vitro effects of eIF1A on Ago2-mediated RNA cleavage. eIF1A or the indicated mutants were incubated with Ago2, synthetic let-7a and 5′- 32 P end-labelled HMGA2 3′-UTR mutants. RNAs were analysed by northern blot and autoradiographs analyses. ( c ) Statistical analyses of three independent in vitro assays in b . ( d ) Western blot assays of effects of eIF1A and eIF1A (K56A) mutant on GFP-let-7 reporter expression. Ago2, eIF1A or eIF1A (K56A) were transiently overexpressed in HEK293 cells stably expressing reporter GFP-let-7. ( e )The expression ratio between tubulin and GFP reporter in the same gel were calculated. Intact (100%) RISC activity was considered in control cells. The relative RISC activities under overexpression conditions of the indicated genes or mutants were obtained by comparison with the control. ( f ) Relative GFP reporter mRNAs in d by quantitative real-time PCR (qPCR). ( g ) Western blot assays of zebrafish c-Myb in the indicated zebrafish groups at 28 h.p.f. (control, eif1axb MO (62.5 μM, 1 nl), eif1axb MO (62.5 μM, 1 nl) plus human eIF1A (heIF1A) (mRNA, 1 μg μl −1 , 1,000 pl) and eif1axb MO (62.5 μM, 1 nl) plus heIF1A (K56A) mutant (mRNA, 1 μg μl −1 , 1,000 pl)). Proteins were extracted from >10 zebrafish per group. ( h ) Relative c-Myb mRNAs in each group in g by qPCR. Total RNAs were extracted from >10 zebrafish per group. ( i ) Taqman PCR assays of relative zebrafish miR-126 (dre-miR-126) in each group in g . Total RNAs were extracted from >10 zebrafish per group. In all statistical comparisons, three independent experiments were performed (mean±s.d., n =3 experiments, Student’s t -test). *** P <0.01. Full size image eIF1A promotes Ago2-mediated miRNA-guided RNAi in vivo To further evaluate the roles of eIF1A on Ago2-mediated RNAi in an animal model, we employed zebrafish. Both zebrafish paralogues eIF1AXa and eIF1AXb interact with Ago2 ( Supplementary Fig. 4a,b ). eif1axb mRNA level is much higher (>25-fold) than that of eif1axa in the developing zebrafish ( Supplementary Fig. 4c,d ), therefore we focused on eif1axb here. We employed a lower dosage of eif1axb Morpholino (MO, 62.5 μM, 1 nl), which does not significantly affect zebrafish phenotypes at 18 h.p.f. (hours post fertilization) and 48 h.p.f. ( Supplementary Fig. 4e,f ). Previous studies reported that miR-126 targets c-Myb and suppresses c-Myb expression in zebrafish [37] . We next examined whether eIF1A plays a role in Ago2-mediated miR-126-guided c-Myb suppression in zebrafish at 28 h.p.f. Zebrafish treated with eif1axb MO (62.5 μM, 1 nl) showed increased c-Myb in comparison with the control group ( Fig. 4g ). Zebrafish with treatment of eif1axb MO (62.5 μM, 1 nl) plus human eIF1A (heIF1A, 1 μg μl −1 mRNA, 1 nl) presented decreased c-Myb levels compared with the group treated with only eif1axb MO (62.5 μM, 1 nl). In contrast, zebrafish treated with human eIF1A K56A (1 μg μl −1 mRNA, 1 nl) and eif1axb MO (62.5 μM, 1 nl) show increased c-Myb ( Fig. 4g ). In addition, heIF1A K56A increased c-Myb mRNA accumulation in zebrafish ( Fig. 4h ), indicating that interfering with eIF1A–Ago2 interaction impairs the miR-126-mediated suppression of c-Myb expression in zebrafish, even though the level of miR-126 remaining is not significantly decreased under these conditions ( Fig. 4i ). These results demonstrated that the eIF1A–Ago2 complex promotes miR-126 RISC activities in vivo . Overall, the above results demonstrate that eIF1A augments Ago2-mediated miRNA-guided RNAi both in vitro and in vivo . eIF1A stimulates miR-451 biogenesis in vitro and in vivo Ago2 is important for Dicer-independent generation of mature miR-451, a miRNA that regulates erythropoiesis [14] , [15] , [16] . We therefore investigated whether eIF1A is involved in Ago2-mediated DICER-independent miRNA biogenesis. In vitro analyses of eIF1A/Ago2-dependent cleavage of pre-miR-451 showed that reactions with eIF1A or eIF1A mutants, but without Ago2, displayed no pre-miR-451 cleavage ( Fig. 5a ). In the presence of Ago2, however, eIF1A enhances pre-miR-451 cleavage in a dose-dependent manner ( Fig. 5a,b ). In contrast, the point mutation of V55A, K56A or K67A impaired the activity of Ago2 in this assay ( Fig. 5a,b ). These results suggest that eIF1A forms a complex with Ago2 to facilitate pre-miR-451cleavage. In northern blot assays, eIF1A mutants (V55A, K56A or K67A) in stable HEK293 cells consistently decreased the production or accumulation of mature miR-451 in comparison with wild-type eIF1A ( Fig. 5c ). Importantly, the level of miR-144—which is processed from the same precursor transcript as miR-451 (refs 14 , 15 )—remained unchanged ( Fig. 5c ). These results suggest that eIF1A promotes Ago2-dependent miR-451 biogenesis in human cells in vitro . While the levels of miRNA-451 increased during development from 24 to 56 h.p.f. in wild-type zebrafish, eif1axb knockdown led to decreased miR-451production ( Fig. 5d ). Human eIF1A (1 μg μl −1 mRNAs, 1 nl) could rescue miR-451 production in eif1axb knockdown zebrafish ( Fig. 5d ). In contrast, heIF1A K56A failed to rescue miR-451 production during zebrafish development ( Fig. 5d ), indicating that eIF1A–Ago2 interaction plays a role in miR-451 biogenesis in vivo . Importantly, eif1axb knockdown does not decrease miR-144 production, indicating that eIF1A does not affect Ago2-independent miRNA production ( Fig. 5d ). These results demonstrated that eIF1A forms a complex with Ago2 and augments Ago2-dependent miR-451 biogenesis in zebrafish. 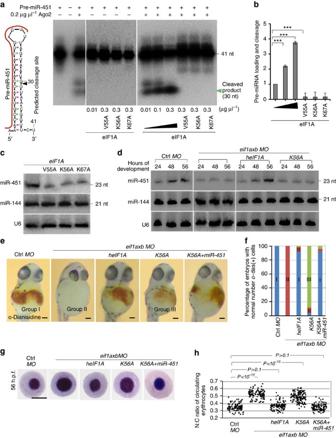Figure 5: eIF1A augments miR-451 biogenesis. (a)In vitroactivity of eIF1A in Ago2-mediated cleavage of 5′-32P end-labelled synthetic pre-miR-451. RNAs were analysed by northern blotting and autoradiographs analyses. (b) Statistical analyses of the data ina. Data of three independent experiments were shown (mean±s.d.,n=3, Student’st-test). (c) Northern blot assays show the effects of eIF1A mutants on miR-451 biogenesis in HEK293 cells. Total RNAs were extracted from stable HEK293 cells expressing Flag-eIF1A and Flag-eIF1A mutants. Signals show mature miR-451 and miR-144 levels with U6 as a loading control. (d) Northern blot assays show the effects of eIF1A(K56A) mutant on miR-451 generation in the developing zebrafish. Total RNAs were extracted from zebrafish with/without treatments of control MO,eif1axbMO (62.5 μM, 1 nl),eif1axbMO (62.5 μM, 1 nl) plus heIF1A (mRNA, 1 μg μl−1, 1 nl),eif1axbMO (62.5 μM, 1 nl) plus heIF1A (K56A) (mRNA, 1 μg μl−1, 1 nl). (e) Haemoglobin (brown) was visualized by the oxidation of o-dianisidine (o-das) in zebrafish at 48 h.p.f. Haemoglobinized cells accumulate in wild-type (group I) and are reduced ineif1axbMO-injected embryos (group II). Human eIF1A, but not K56A mutant (group III, with less haemoglobinized cells), rescues haemoglobinized cells ineif1axbMO-injected zebrafish, while miR-451 spares K56A-caused rescue defects. Scale bar, 100 μm. (f) Percentage of embryos with haemoglobinized cells in zebrafish. Control group (n=40).eif1axbMO injection (n=42). Human eIF1A (n=35), but not K56A mutant (n=35), increased the percentage of embryos with normal haemoglobinized cells, while miR-451 (n=31) suppresses the decreased percentage by K56A mutant (P<0.001). (g) Erythrocytes stained with May-Grünwald/Giemsa are representative of the mean of each group at 56 h.p.f. Scale bar, 5 μm. (h) Scatterplot of the nuclear cytoplasmic ratio (N:C) for each group as a readout of erythrocyte maturation (Wilcoxon rank-sum test after Bonferroni correction,P<10−15). Human eIF1A (n=120 erythrocytes), but not K56A mutant (n=145), rescued erythrocyte maturation impaired byeif1axbMO injection, while miR-451(n=118) spares distribution difference in the heIF1A(K56A) mutant group. ***P<0.01. Figure 5: eIF1A augments miR-451 biogenesis. ( a ) In vitro activity of eIF1A in Ago2-mediated cleavage of 5′- 32 P end-labelled synthetic pre-miR-451. RNAs were analysed by northern blotting and autoradiographs analyses. ( b ) Statistical analyses of the data in a . Data of three independent experiments were shown (mean±s.d., n =3, Student’s t -test). ( c ) Northern blot assays show the effects of eIF1A mutants on miR-451 biogenesis in HEK293 cells. Total RNAs were extracted from stable HEK293 cells expressing Flag-eIF1A and Flag-eIF1A mutants. Signals show mature miR-451 and miR-144 levels with U6 as a loading control. ( d ) Northern blot assays show the effects of eIF1A(K56A) mutant on miR-451 generation in the developing zebrafish. Total RNAs were extracted from zebrafish with/without treatments of control MO, eif1axb MO (62.5 μM, 1 nl), eif1axb MO (62.5 μM, 1 nl) plus heIF1A (mRNA, 1 μg μl −1 , 1 nl), eif1axb MO (62.5 μM, 1 nl) plus heIF1A (K56A) (mRNA, 1 μg μl −1 , 1 nl). ( e ) Haemoglobin (brown) was visualized by the oxidation of o-dianisidine (o-das) in zebrafish at 48 h.p.f. Haemoglobinized cells accumulate in wild-type (group I) and are reduced in eif1axb MO-injected embryos (group II). Human eIF1A, but not K56A mutant (group III, with less haemoglobinized cells), rescues haemoglobinized cells in eif1axb MO-injected zebrafish, while miR-451 spares K56A-caused rescue defects. Scale bar, 100 μm. ( f ) Percentage of embryos with haemoglobinized cells in zebrafish. Control group ( n =40). eif1axb MO injection ( n =42). Human eIF1A ( n =35), but not K56A mutant ( n =35), increased the percentage of embryos with normal haemoglobinized cells, while miR-451 ( n =31) suppresses the decreased percentage by K56A mutant ( P <0.001). ( g ) Erythrocytes stained with May-Grünwald/Giemsa are representative of the mean of each group at 56 h.p.f. Scale bar, 5 μm. ( h ) Scatterplot of the nuclear cytoplasmic ratio (N:C) for each group as a readout of erythrocyte maturation (Wilcoxon rank-sum test after Bonferroni correction, P <10 −15 ). Human eIF1A ( n =120 erythrocytes), but not K56A mutant ( n =145), rescued erythrocyte maturation impaired by eif1axb MO injection, while miR-451( n =118) spares distribution difference in the heIF1A(K56A) mutant group. *** P <0.01. Full size image eIF1A modulates miR-451-mediated erythrocyte maturation Recent studies have reported that miR-451 plays an important role in erythrocyte maturation in zebrafish [15] , [38] , [39] . Consistent with a role for eIF1A in miR-451 biogenesis, injection of human eIF1A mRNAs (1 μg μl −1 , 1 nl, n =35 embryos), but not mRNAs encoding human eIF1A K56A (1 μg μl −1 , 1 nl, n =35), rescues the reduced haemoglobinized cells in zebrafish with eif1axb gene knockdown ( Fig. 5e,f ). Importantly, miR-451 (0.2 μg μl −1 , 1 nl, n =31) partly compensated the decrease in haemoglobinized cells in zebrafish treated with eif1axb knockdown or heIF1A K56A ( Fig. 5e,f ). Furthermore, heIF1A ( n =120 erythrocytes), but not heIF1A K56A mutant ( n =145 erythrocytes), rescued erythrocyte maturation in zebrafish with eif1axb knockdown. Notably, miR-451 (0.2 μg μl −1 , 1 nl, n =118 erythrocytes) rescued erythrocyte maturation delay caused by heIF1A K56A expression ( Fig. 5g,h ). These results demonstrate that eIF1A modulates miR-451 production in zebrafish. Taken together, our data demonstrate that eIF1A forms a complex with Ago2 and promotes Ago2-mediated miRNA-guided RNAi and Ago2-dependent Dicer-independent miRNA biogenesis. Ago2-mediated miRNA biogenesis and processing are essential for the development in eukaryotes. We found that eIF1A directly binds to Ago2 in an RNA-independent manner, and plays a role in both Ago2-mediated miRNA-guided RNAi and miRNA biogenesis ( Fig. 6 ). Using biochemistry and NMR analyses, we demonstrated that the MID domain of Ago2 binds to the GD of eIF1A. eIF1A promotes Ago2-mediated RNAi and miR-451 biogenesis in vitro and in vivo . eIF1A augments erythrocyte maturation in zebrafish through mediating miR-451 surveillance. The previously unrecognized roles of eIF1A in Ago2-mediated miRNA processes identified here provide insights into the understanding of the mechanisms of miRNA-guided RNAi and miRNA biogenesis. 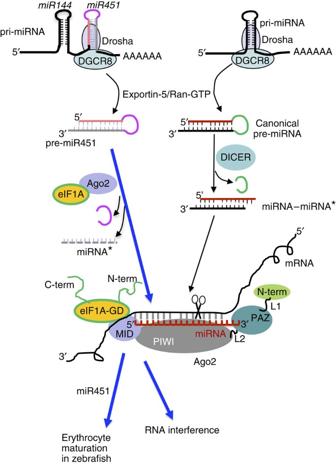Figure 6: Schematic diagram for eIF1A functions in Ago2-dependent miR-451 biogenesis, RNA interference and erythrocyte maturation in zebrafish. The primary miRNA (priRNA) is cleaved by Drosha-DGCR8 pathways to generate pre-miRNA within the nucleus. Exportin-5 in complex with Ran-GTP exports the pre-miRNA to the cytoplasm, where the pre-miRNA is bound by DICER to form a RISC loading complex that includes Ago2. In the canonical miRNA biogenesis pathway, DICER removes the terminal loop region to yield the mature miRNA. The pre-miR-451 is loaded directly onto Ago2 and sliced on the 3′-hairpin arm. The miR-144 biogenesis is DICER dependent. The globular domain (GD) of eIF1A directly binds to the MID domain of Ago2 and forms an eIF1A–Ago2 complex promoting Ago2-mediated RNAi and miR-451 biogenesis. The MID domain of Ago2 binds to the GD of eIF1A and does not impair eIF1A functions in translation initiation. The 5′-term of guide strand of miRNA–miRNA* duplex is docked onto a pocket with residues mainly from the MID domain. The long and structured mRNAs are scanned by RISCs to recognize seed regions in miRNAs. After a perfect or imperfect complementary guide with miRNAs, mRNAs are nicked by the PIWI domain resulting in RNAi. eIF1A augments Ago2-mediated RNAi, miR-451 production and erythrocyte maturation. Black arrows are from previous reports of other groups14,15,43; blue arrows are from this study. Figure 6: Schematic diagram for eIF1A functions in Ago2-dependent miR-451 biogenesis, RNA interference and erythrocyte maturation in zebrafish. The primary miRNA (priRNA) is cleaved by Drosha-DGCR8 pathways to generate pre-miRNA within the nucleus. Exportin-5 in complex with Ran-GTP exports the pre-miRNA to the cytoplasm, where the pre-miRNA is bound by DICER to form a RISC loading complex that includes Ago2. In the canonical miRNA biogenesis pathway, DICER removes the terminal loop region to yield the mature miRNA. The pre-miR-451 is loaded directly onto Ago2 and sliced on the 3′-hairpin arm. The miR-144 biogenesis is DICER dependent. The globular domain (GD) of eIF1A directly binds to the MID domain of Ago2 and forms an eIF1A–Ago2 complex promoting Ago2-mediated RNAi and miR-451 biogenesis. The MID domain of Ago2 binds to the GD of eIF1A and does not impair eIF1A functions in translation initiation. The 5′-term of guide strand of miRNA–miRNA* duplex is docked onto a pocket with residues mainly from the MID domain. The long and structured mRNAs are scanned by RISCs to recognize seed regions in miRNAs. After a perfect or imperfect complementary guide with miRNAs, mRNAs are nicked by the PIWI domain resulting in RNAi. eIF1A augments Ago2-mediated RNAi, miR-451 production and erythrocyte maturation. Black arrows are from previous reports of other groups [14] , [15] , [43] ; blue arrows are from this study. Full size image Interestingly, point mutation of K56A in eIF1A leads to dissociation of eIF1A–Ago2 interaction. The eIF1A (K56A) mutant does not impair translation initiation. In contrast, eIF1A(K56A) impairs Ago2-mediated miRNA-guided RNAi and Ago2-dependent miR-451 production in vitro and in zebrafish in vivo . Consistently, miR-451 partly reverts reduced haemoglobinization and delayed maturation of erythrocytes in eif1axb knockdown zebrafish with overexpressed heIF1A (K56A). These data demonstrate that eIF1A–Ago2 interaction promotes Ago2-mediated RNAi and miRNA production but does not compromise eIF1A functions in translation initiation. Recently, Ameres et al . [40] , Cheloufi et al . [14] and Cifuentes et al . [15] have reported that recombinant Ago2 is sufficient for slicer activity with large quantities of RNA fragments in RNAi and miR-451 processing in vitro . These data elegantly evidenced that Ago2 is a central effector of miR-451 generation and RNAi processes. On the other hand, many studies demonstrated that the Ago2-centred RISC complex is necessary for efficient RNAi activity with long and/or structured mRNAs and miR-451 processing in vivo [23] , [41] . It is possible that other components in RISC are needed to resolve the mRNA secondary structure, to scan the long and/or structured mRNAs for recognition of miRNA seed regions in low abundance and to generate mature miR-451. Currently, the component list of RISC is increasing. Here we show that eIF1A directly binds to Ago2 and augments miR-451 biogenesis and RNAi processes, suggesting that eIF1A is an important but previously unrecognized factor of RISC. The MID domain of Ago2 is essential for miRNA docking in RISC-mediated RNAi and pre-miR-451 loading in Dicer-independent miR-451 biogenesis. Here, we found that eIF1A directly binds to the MID domain of Ago2, and eIF1A promotes miRNA-guided RNAi and miR-451 generation. Our findings reveal that eIF1A directly interacts with Ago2 and augments Ago2-mediated miRNA-guided RNAi and DICER-independent miRNA biogenesis. The newly identified eIF1A–Ago2 complex together with its functions in miRNA processes provides insights in understanding how Ago2 mediates miRNA processes in translation, development and diseases. Plasmids, antibodies and reagents Constructs of human Flag-HA-Ago1(10820), Ago2 (10822), Ago3 (10823) and Ago4 (10824) were obtained from Addgene. The complementary DNAs (cDNAs) of human eIF1A were PCR-amplified from HEK293 cDNAs. Human eIF1A was inserted into NotI/EcoRI sites of the pIRESneo vector. Mutants of eIF1A: ND (25 ∼ 144 aa, amino acid), CD (1 ∼ 114 aa), GD (25 ∼ 114 aa) were generated by PCR and inserted into NotI/EcoRI sites of the pIRESneo vector encoding an N terminus with Flag-HA. Monoclonal anti-Flag (#8146S) antibody (20 μl for the immunoprecipitation assay), monoclonal anti-HA antibody (6E2, 2367S, 20 μl for the immunoprecipitation assay) and monoclonal anti-GFP antibody (#2956S, 20 μl for the immunoprecipitation assay, 1:1,000 dilution for the western blot assay) and anti-β-Tubulin (2146S, 1:1,000 dilution for the western blot assay) were ordered from Cell Signaling. Monoclonal anti-eIF1A antibody (Ab172623, 20 μl for the immunoprecipitation assay; 1:1,000 dilution for the western blot assay), monoclonal anti-human Ago2 antibody (ab57113, used to detect human and zebrafish Ago2, 1:1,000 dilution for the western blot assay, 20 μl for the immunoprecipitation assay) and polyclonal anti-actin (ab1801, for zebrafish actin detection with 1:1,000 dilution for the western blot assay) were bought from Abcam. Polyclonal anti-Ago1 (SAB4200065, 1:1,000 dilution for the western blot assay) and Ago3 (SAB4200112, 1:1,000 dilution for the western blot assay) antibodies were purchased from Sigma. Polyclonal anti-Ago4 antibody (MABE139, 1:1,000 dilution for the western blot assay) was ordered from Millipore. Ribonuclease A was ordered from Sigma. Benzonase nuclease was ordered from VWR. HEK293 (CRL-1573), HeLa (CCL-2) and T98G (CRL-1690) cells were ordered from ATCC. SilverXpress Silver Staining Kit was purchased from Invitrogen. The CellTiter-Glo Luminescent Cell Viability Assay Kit was bought from Promega. Immunoprecipitation, MS and western blot assays The stable HEK293 cell line expressing Flag-HA (as a control) or Flag-HA-Ago2 were lysed with lysis buffer containing 20 mM Tris HCl pH 7.4, 137 mM NaCl, 10% glycerol, 1% NP-40, EDTA-free protease inhibitor (Roche) followed by 10 μg ml −1 ribonuclease A treatment (25 °C, 1 h). The Ago2-interacted proteins were immunoprecipitated by anti-HA monoclonal antibodies (Cell Signaling, 2367S, 20 μl for the immunoprecipitation assay) immobilized to Dyna beads. The purified proteins were analysed by silver staining and mass spectrometry (MS) via liquid chromatography-MS/MS on an LTQ Orbitrap Velos mass spectrometer (Thermo Scientific, Germany) equipped with a Thermo Fisher Scientific nanospray source, an Agilent 1,100 Series binary HPLC pump and a Famos autosampler. The spectral data were searched with SEQUEST against a database containing the human International Protein Index protein sequence database: ( http://www.ebi.ac.uk/IPI/ ) together with the reversed complement. eIF1A was transiently overexpressed in stable HEK293 cell lines expressing Agos (Ago1 ∼ 4). The cell lysates were treated with 10 μg ml −1 ribonuclease A (25 °C, 1 h). Immunoprecipitated proteins by anti-eIF1A monoclonal antibodies (Abcam, Ab172623, 20 μl for immunoprecipitation assay) were analysed by western blotting with anti-Agos (1 ∼ 4) antibodies (monoclonal anti-Ago2 antibodies, Abcam, ab57113, 1:1,000 dilution; polyclonal anti-Ago1/3, Sigma, SAB4200065, SAB4200112, 1:1,000 dilution); Ago4 Millipore, MABE139, 1:1,000 dilution) antibodies in immunoblotting. Expression and purification of eIF1A and Ago2 fragments The cDNA for the MID domain of human Ago2 (His-Sumo-tagged) was provided by Bhushan Nagar (McGill University). Human eIF1A and mutants of eIF1A-ND/-CD/-GD were inserted into EcoRI/NotI sites of pGEX-4E-1 vectors with GST fusion at the N-terminal. Human Ago2 (full length) and fragments of L1 (172 ∼ 227 aa), PAZ (227 ∼ 349 aa), MID (432 ∼ 575 aa) and PIWI (590 ∼ 816 aa) were inserted into NdeI/BamHI sites of a pET-6H2 vector. His-tagged proteins expressed in BL21(DE3) cells were extracted by sonication with lysis buffer (50 mM Tris, 350 mM NaCl, 10 mM imidazole, pH 8.0, 20 μM Benzonase nuclease, 10 μg ml −1 RNase A, 100 μg ml −1 lysozyme, 2% NP-40, 0.05% β-mercaptoethanol and protease inhibitor) followed by Ni-agarose resin (Qiagen) purification. GST-tagged proteins expressed in BL21(DE3) cells were extracted by MagneGST Protein Purification System (Promega) or Pierce Glutathione Magnetic Beads (Thermo Scientific). GST pull-down assays Escherichia coli -expressed GST-tagged human eIF1AX (known as eIF1A), or GD (25 ∼ 114 aa), or ND (25 ∼ 144 aa) or CD (1 ∼ 114 aa) were purified by GST pull-down assays (#88822, Thermo Scientific) with glutathione magnetic beads from pre-cleared cell lysates of HEK293 cells stably expressing HA-Ago2 in the presence of 10 μg ml −1 ribonuclease A treatment. Western blot assays were performed with anti-Ago2 monoclonal antibodies (Abcam, ab57113, 1:1,000 dilution). For the Ago2 domain screening assays, E. coli expressed His-tagged L1, PAZ, Sumo-MID, PIWI domains and Sumo, which were purified by Ni-NTA resin, were performed GST pull-down assays with E. coli expressed GST-eIF1A. Western blot assays were performed with anti-His monoclonal antibodies (Cell Signaling, #2366S, 1:1,000 dilution). Nuclear Magnetic Resonance (NMR) titrations BL21(DE3) bacterial cells harbouring His-SMT3, His-SMT3-tagged MID(432 ∼ 575 aa) and His-tagged eIF1A were grown in either LB or minimal media containing 15 N ammonium chloride. The resulting cell pellets were lysed by sonication or French press with lysis buffer (50 mM Tris, 350 mM NaCl, 10 mM imidazole, pH 8.0, 20 μM Benzonase nuclease, 10 μg ml −1 RNase A, 100 μg ml −1 lysozyme, 2% NP-40, 0.05% β-mercaptoethanol and protease inhibitor). The soluble proteins were loaded onto a Ni-agarose resin (Qiagen) and proteins were eluted with Ni-elution buffer (50 mM Tris, 350 mM NaCl, 350 mM imidazole, pH 8.0). Purified proteins in Ni-elution buffer were further purified by size-exclusion chromatography using a S75 column and eluting with HEPES buffer (20 mM HEPES, 150 mM NaCl, 0.5 mM TCEP, pH 7.2). The heteronuclear single-quantum coherence measurements were carried out on a Bruker 500 MHz and Varian 600 MHz instrument each equipped with a cryogenically cooled probe. The data were processed using NMRPipe and visualized using CARA. The molar ratios of 15 N-eIF1A:SMT3-MID at 1:1 were analysed in this study and the concentration of 15 N-eIF1A was at 200 μM. Similarly 15 N-SMT3-MID was held at concentration of 200 μM and unlabelled eIF1A was titrated at a molar ratio of 1:1. Ago2-mediated RNAi and miR-451 biogenesis in vitro assays Target miRNA cleavage analyses [14] , [15] for Ago2 proteins were performed. Briefly, overexpressed HA-Ago2, HA-eIF1A and HA-eIF1A mutant (V55A, K56A and K67A) proteins were purified with anti-HA antibodies and Dyna beads (Invitrogen) from HEK293 cells via native methods. For the in vitro miRNA mediated RNA slicing assays, 100 μM let-7a (Dharmacon) and linearized 5 μM 5′- 32 P end-labelled synthetic HMGA2 3′-UTR mutant (IDT) were performed Ago2 cleavage analyses were incubated with eIF1A in a series of concentrations (0.01, 0.1 and 0.3 μg μl −1 ) or eIF1A mutants (0.3 μg μl −1 ) at 37 °C for 4 h in a 10-μl reaction volume. The reaction contained 3 μg of yeast tRNAs, 25 mM HEPES-KOH pH 7.5, 50 mM potassium acetate, 5 mM magnesium acetate, 5 mM dithiothreitol (DTT), 0.1 μl (1 μg μl −1 ) native HEK293 cell lysates, 100 μM let-7a and linearized 5 μM 5′- 32 P end-labelled synthetic HMGA2 3′-UTR mutant, with/without 0.2 μg μl −1 Ago2. For the in vitro pre-miR-451 cleavage analysis, 5 μM of 5′- 32 P end-labelled synthetic pre-miR-451 (Dharmacon) and 0.2 μg μl −1 Ago2 were incubated with eIF1A in a series of concentrations (0.01, 0.1 and 0.3 μg μl −1 ), or eIF1A mutants (V55A, K56A and K67A) (0.3 μg μl −1 ) in a 10-μl reaction volume at 37 °C for 4 h. The reaction contained 3 μg of yeast tRNAs, 25 mM HEPES-KOH pH 7.5, 50 mM potassium acetate, 5 mM magnesium acetate, 5mM DTT and 0.1 μl (1 μg μl −1 ) native HEK293 cell lysate. The ethanol-precipitated RNAs were analysed in 4 ∼ 20% Mini-PROTEAN TBE Precast Gel (Bio-Rad). The gel was quantified by Phosphorimager analyses. Endogenous miRNA-guided RISC activity assays To read miRNA-guided RISC activity, pcDNA-GFP- let-7 (complementary sequence of miRNA let-7 , 5′-AACTATACAACCTACTACCTCA-3′) was generated in HEK293 cells as previously described [36] . The pcDNA-GFP- let-7 was transfected into HEK293 cells followed by 1.6 mg ml −1 G418 selection for 2 weeks. The resistant colonies were propagated into stable cell lines. For the let-7 RISC activity assay, 2 μg of expression constructs were transfected into 5 × 10 5 cells of the GFP-reporter stable cell lines in six-well plates and the cells were transferred to 10-cm plates after 24 h. After 36 h, total proteins were extracted with standard RIPA buffer together with protease inhibitor (Roche) and total RNAs were extracted using Trizol reagents (Invitrogen). Control MO or 62.5 μM eif1axb MO plus 1 μg μl −1 human eIF1A or mutant mRNAs were injected into one-cell-stage zebrafish embryos. Total RNAs and proteins were isolated at 48 h.p.f. for the analyses of c-Myb proteins and mRNAs. Zebrafish eif1axb knockdown and mRNA microinjection The wild-type AB/C32 -strain zebrafish were used in this study. All the experiments were conducted according to US National Institutes of Health guidelines for animal research and were approved by Harvard Medical Animal Committee. The MO targeting +1 ∼ +25 of eif1axb (5′-CTCCTTTTCCTTTGTTTTTCGGCAT-3′) and control MO (5′-CCTCTTACCTCAGTTACAATTTATA-3′) were obtained from Gene Tools. Zebrafish embryos were injected at the one-cell stage with 1 nl of 250 μM control, 250 μM eif1axa , 250 μM eif1axb , 125 μM eif1axb and combined 125 μM eif1axa+ 125 μM eif1axb MO with a PLI-100 A Pico-Injector. Images were taken at 19, 28 and 45 h.p.f. Total RNAs and proteins were extracted for miRNA, real-time qPCR and western blot assays. Antibodies of anti-Ago2 (ab57113, monoclonal), anti-eIF1A (ab38976, polyclonal) and anti-c-Myb (ab62824, polyclonal) ordered from Abcam were used in zebrafish western blot assays. Antibodies of anti-β-actin (#4967, polyclonal) were ordered from Cell Signaling. The qPCR assays were performed with primers (forward and backward): 5′-GAACGGCATCAAGGTGAACTT-3′ and 5′-GACGACCTCGAGTGAGGTAGTAGGTTGTATA-3′ for GFP-let-7; 5′-AAATCTGGCACCACACCTTCTAC-3′ and 5′-GATAGCACAGCCTGGATAGCAAC-3′ for human β-actin; 5′-GCATCATGGTTCTGAAGACTGG-3′ and 5′-CTTCTGCACCAACTCAATCACC-3′ for c-Myb; 5′-GACCCAGACATCAGGGAGTGAT-3′ and 5′-ATGCCAGATCTTCTCCATGTCA-3′ for zActin; 5′-CCAGGATGTCAAAGCAGATGTC-3′ and 5′-ATGTCGTCATCGTTCTCTCCAA-3′ for eif1axa; 5′-TCATCAAGATGTTGGGAAATGG-3′ and 5′-CCTAGCCTCGTCGGCATTATAC-3′ for eif1axb. Northern blot assays Total RNAs were isolated from HEK293 cells, stable HEK293 cells expressing eIF1A mutants (V55A, K56A or K67A) and developing zebrafish with Trizol (Invitrogen). Twenty-five μg total RNAs were loaded into each well of TBE precast gel (Bio-Rad). Northern blot experiments were performed with semi-dry transfer cell and 5′- 32 P-labelled probes. The mature miR-451- and miR-144-specific probes sequences are: 5′-AACUCAGUAAUGGUAACGGUUU-3′ for miR-451; 5′-AGUACAUCAUCUAUACUGUA-3′ for miR-144. U6 probe: 5′-AAAAAUAUGGAACGCUUCACGAAUUUG-3′ for U6 (probes were ordered from IDT). Taqman real-time PCR Mature miRNA-specific Taqman real-time PCR was performed as per the TaqMan manufacturer instructions (Taqman microRNA reverse transcription Kit, TaqMan Universal Master Mix II, no UNG Mini-Pack and TaqMan Small RNA assay) described with the following sequences: let-7 (5′-UGAGGUAGUAGGUUGUAUAGUU-3′), miR-126 (5′-UCGUACCGUGAGUAAUAAUGC-3′). Data were normalized to let-7 in zebrafish samples and calculated as described by the manufacturer. The s.d. were obtained from three independent experiments. mRNA preparation and rescue analyses The pCS2Flag constructs (pCS2Flag-vector from Addgene, #16331) harbouring genes encoding human eIF1A or eIF1A (K56A) were linearlized with the ApaI restriction enzyme. The mRNAs were prepared using the mMESSAGE mMACHINE SP6 Kit (Invitrogen) following the manufacturer’s instructions. The mRNAs were purified using the RNeasy Plus Mini Kit (Qiagen) with RNase-free H 2 O. Rescue of the eif1axb MO (62.5 μM, 1 nl)-introduced zebrafish was performed by injection of 1,000 pl of a 1-μg μl −1 mRNA-encoding human eIF1A or eIF1A (K56A) into wild-type one-cell-stage zebrafish embryos. Experiments with injection of 1,000 pl of eif1axb MO (62.5 μM) plus 1 μg μl −1 mRNA-encoding human eIF1A (K56A) and 0.2 μg μl −1 miR-451(IDT) were performed. Site-directed mutagenesis The Pfu DNA polymerase-PCR (Pfu-PCR) assays for the site-directed mutagenesis of V55A, K56A and K67A of HA-tagged human eIF1A were performed. Pfu DNA polymerase is an enzyme found in the hyperthermophilic archaeon Pyrococcus furiosus. We used the following primers: V55A: sense: 5′-GCAATGTGTTTCGATGGTGCAAAGAGGTTATGTCACATC-3′; antisense: 5′-GATGTGACATAACCTCTTTGCACCATCGAAACACATTGC-3′; K56A: sense: 5′-GAAGCAATGTGTTTCGATGGTGTAGCGAGGTTATGTCACATCAG-3′; antisense: 5′-CTGATGTGACATAACCTCGCTACACCATCGAAACACATTGCTTC-3′; K67A: sense: 5′-GTCACATCAGAGGAAAATTGAGAGCAAAGGTTTGGATAAATACCTCGG-3′; antisense: 5′-CCGAGGTATTTATCCAAACCTTTGCTCTCAATTTTCCTCTGATGTGAC-3′. The reactions in volume of 10μl of each with sense primers or antisense primers were separately performed pfu-PCR with procedures: (1) 95 °C, 3 min; (2) 95 °C, 20 s; (3) 65 °C 20 s; (4) 72 °C, 5–12 min; 10 cycles (steps 2 ∼ 4); (5) 72 °C, 10 min; (6) 4 °C. Combine the sense reaction and antisense reaction products (total volume of 20 μl for each reaction) and continue pfu-PCR with procedures: (1) 95 °C, 3 min; (2) 95 °C, 20 s; (3) 65 °C 20 s; (4) 72 °C, 5–12 min; 20 cycles (steps 2 ∼ 4); (5) 72 °C, 10 min; (6) 4 °C. The pfu-PCR products were digested with DpnI restriction enzyme (New England Biolabs) at 37 °C for 2 h. The DNAs were transformed into Z-Competent E. Coli Cells-Strain Zymo 5α (Zymo Research). Constructs, which were validated by sequencing, harbouring correct sequences encoding HA-tagged eIF1A (V55A), eIF1A (K56A) and eIF1A (K67A) were used in this study. Polysome profiling Growth medium was aspirated and cells were washed with PBS, recovered in lysis buffer (50 mM HEPES/KOH pH 7.5, 100 mM NH 4 Cl, 25 mM MgCl 2 , 1 mM DTT and 0.5% (w/v) Triton X-100) and passed 6 × through a 27-gauge needle. Insoluble material was removed by a 3- min spin (microcentrifuge, 20,817 r.c.f.). All steps during sample preparation were done on ice or at 4 °C. Approximately 100 μl of the lysates (corresponding to ≈2 × 10 6 cells) were loaded onto linear sucrose density gradients (10–40% (w/v) sucrose in lysis buffer) and centrifuged for 2 h at 40,000 r.p.m. (SW40 rotor, Beckman Coulter) at 4 °C. The gradients were fractionated on a Piston Gradient Fractionator (BioComp Instruments, Fredericton, Canada) and ribosome profiles were recorded at 260 nm. In vitro translation assays The dicistronic reporter construct, containing the Renilla luciferase sequence after the 5′-UTR followed by the CrPV IRES and the firefly luciferase sequence, has been previously described [42] . The reporter construct plasmid was linearized with BamHI (New England Biolabs) and transcribed in vitro with an ARCA cap and poly(A)-tailed using the mMessage Machine T7 Ultra Kit (Ambion). The mRNAs were purified using the RNeasy Plus Mini Kit (Qiagen) with RNase-free H 2 O. Human eIF1A and mutants (V55A, K56A and K67A, with anti-Flag antibodies, 0.15 mg ml −1 , 2 μl per reaction) were purified using Dyna beads (Invitrogen) from HEK293 cells with transient transfection of plasmids encoding Flag-tagged eIF1A and eIF1A mutants. In vitro translation reactions (50 μl per reaction) were carried out using Rabbit Reticulocyte Lysate (Promega, 35 μl per reaction) with 2 mM magnesium acetate and 60 mM potassium acetate, which was incubated at 30 °C for 100 min. Translation of the reporter genes was measured using the Dual-Glo luciferase assay (Promega). Three independent experiments were performed. O-dianisidine staining O-dianisidine (Sigma) solution at 0.7 mg ml −1 was prepared in fresh ethanol and protected from exposure to light. The staining solution was prepared by mixing 2 ml of water, 2 ml of 0.7-mg ml −1 o-dianisidine solution, 0.5 ml of 100 mM sodium acetate and 100 μl of 3% hydrogen peroxide. Phenylthiourea (PTU)-treated 48-h.p.f. embryos were transferred to 12-well plates and 1 ml of the staining solution was added. Stained embryos were kept in the dark for 15 min, washed three times with 1 × PBS and fixed with 4% paraformaldehyde. May-Grünwald/Giemsa staining Erythrocyte collection from 20 zebrafish (56 h.p.f.) of each group was performed by cutting the zebrafish tails. Circulating erythrocytes were collected with 1 × PBS with 10% FBS with cytospin. The erythrocytes on slides were stained with May-Grünwald/Giemsa solutions (Polysciences), imaged and photographed using a Nikon 80i Upright Microscope. The pixel area of the nucleus and cytoplasm was quantified for 100–145 cells per sample in three independent experiments using ImageJ software, and the nuclear:cytoplasmic ratio was calculated for each cell. Image acquisition In o-dianisidine staining assays, stained embryos were imaged and photographed using a Leica M80 microscope with a Nikon D200 digital camera using an adjustable flash system. Erythrocytes with May-Grünwald/Giemsa staining were imaged using the Nikon 80i Upright Microscope in the Nikon Image Center at Harvard Medical School. Fluorescence and/or 4′,6-diamidino-2-phenylindole-stained images were taken with a Nikon Ti Inverted Fluorescence microscope with Perfect Focus System in the Nikon Image Center at Harvard Medical School. Images of zebrafish embryos were taken by a Leica M80 microscope using a Nikon D200 digital camera. Statistical analyses All statistical experimental data are presented as mean±s.d. ( n =3 or more). P value was determined by the Student’s t -test (tail=2). *** P <0.01. How to cite this article : Yi, T. et al . eIF1A augments Ago2-mediated Dicer-independent miRNA biogenesis and RNA interference. Nat. Commun . 6:7194 doi: 10.1038/ncomms8194 (2015).